A solid with a hierarchical tetramodal micro-meso-macro pore size distribution Porous solids have an important role in addressing some of the major energy-related problems facing society. Here we describe a porous solid, α-MnO 2 , with a hierarchical tetramodal pore size distribution spanning the micro-, meso- and macro pore range, centred at 0.48, 4.0, 18 and 70 nm. The hierarchical tetramodal structure is generated by the presence of potassium ions in the precursor solution within the channels of the porous silica template; the size of the potassium ion templates the microporosity of α-MnO 2 , whereas their reactivity with silica leads to larger mesopores and macroporosity, without destroying the mesostructure of the template. The hierarchical tetramodal pore size distribution influences the properties of α-MnO 2 as a cathode in lithium batteries and as a catalyst, changing the behaviour, compared with its counterparts with only micropores or bimodal micro/mesopores. The approach has been extended to the preparation of LiMn 2 O 4 with a hierarchical pore structure. Porous solids have an important role in addressing some of the major problems facing society in the twenty-first century, such as energy storage, CO 2 sequestration, H 2 storage, therapeutics (for example, drug delivery) and catalysis [1] , [2] , [3] , [4] , [5] , [6] , [7] , [8] . The size of the pores and their distribution directly affect their ability to function in a particular application [2] . For example, zeolites are used as acid catalysts in industry, but their micropores impose severe diffusion limitations on the ingress and egress of the reactants and the catalysed products [9] . To address such issues, great effort is being expended in preparing porous materials with a bimodal (micro and meso) pore structure by synthesizing zeolites or silicas containing micropores and mesopores [10] , [11] , [12] , [13] , [14] , [15] , [16] , [17] , or microporous metal–organic frameworks with ordered mesopores [18] . Among porous solids, porous transition metal oxides are particularly important, because they exhibit many unique properties due to their d -electrons and the variable redox state of their internal surfaces [8] , [19] , [20] , [21] , [22] . Here we describe the first solid (α-MnO 2 ) possessing hierarchical pores spanning the micro, meso and macro range, centred at 0.48, 4.0, 18 and 70 nm. The synthesis method uses mesoporous silica as a hard template. Normally such a template generates a mesoporous solid with a unimodal [23] , [24] , [25] , [26] , [27] , [28] , [29] , [30] , [31] or, at most, a bimodal pore size distribution [32] , [33] , [34] , [35] , [36] , [37] , [38] . By incorporating K + ions in the precursor solution, within the silica template, the K + ions act bifunctionally: their size templates the formation of the micropores in α-MnO 2 , whereas their reactivity with silica destroys the microporous channels in KIT-6 comprehensively, leading to the formation of α-MnO 2 containing large mesopores and, importantly, macropores, something that has not been possible by other methods. Significantly, this is achieved without destroying the silica template by alkaline ions. The effect of the tetramodal pore structure on the properties of the material is exemplified by considering their use as electrodes for lithium-ion batteries and as a catalyst for CO oxidation and N 2 O decomposition. The novel material offers new possibilities for combining the selectivity of small pores with the transport advantages of the large pores across a wide range of sizes. We also present results demonstrating the extension of the method to the synthesis of LiMn 2 O 4 with a hierarchical pore structure. Composition of tetramodal α-MnO 2 The composition of the synthesized material was determined by atomic absorption analysis and redox titration to be K 0.08 MnO 2 (the K/Mn ratio of the precursor solution was 1/3). The material is commonly referred to as α-MnO 2 , because of the small content of K + [19] . N 2 sorption analysis of tetramodal α-MnO 2 The tetramodal α-MnO 2 shows a type IV isotherm ( Fig. 1a ). The pore size distribution ( Fig. 1b ) in the range of 0.3–200 nm was analysed using the density functional theory (DFT) method applied to the adsorption branch of the isotherm [39] , [40] , [41] , [42] , as this is more reliable than analysing the desorption branch [43] ; note that this is not the DFT method used in ab initio electronic structure calculations. Plots were constructed with vertical axes representing ‘incremental pore volume’ and ‘incremental surface area’. Large (macro) pores can account for a significant pore volume while representing a relatively smaller surface area and vice versa for small (micro) pores. Therefore, when investigating a porous material with a wide range of pore sizes, for example, micropore and macropore, the combination of surface area and pore volume is essential to determine the pore size distribution satisfactorily ( Fig. 1b ). Considering both pore volume and surface area, significant proportions of micro-, meso- and macropores are evident, with distinct maxima centred at 0.70, 4.0, 18 and 70 nm. To probe the size of the micropores more precisely than is possible with DFT, the Horvath–Kawazoe pore size distribution analysis was employed [44] . A single peak was obtained at 0.48 nm ( Fig. 1c ), in good accord with the 0.46-nm size of the 2 × 2 channels of α-MnO 2 (refs. 19 , 21 ). The relatively small Brunauer–Emmett–Teller (BET) surface area of tetramodal α-MnO 2 (79–105 m 2 g −1 ; Supplementary Table S1 ) compared with typical surface areas of mesoporous metal oxides (90–150 m 2 g −1 ) [45] is due to the significant proportion of macropores (which have small surface areas) and relatively large (18 nm) mesopores—a typical mesoporous metal oxide has only 3–4 nm pores. 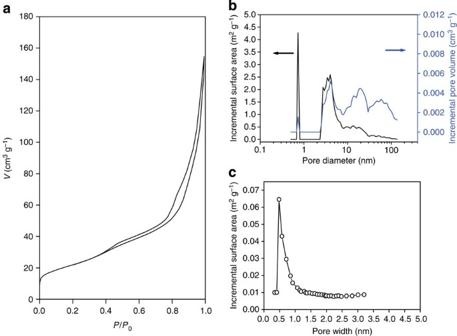Figure 1: N2sorption analysis of tetramodal α-MnO2. (a) N2adsorption–desorption isotherms, (b) DFT pore size distribution and (c) Horvath–Kawazoe pore size distribution from N2adsorption isotherm for tetramodal α-MnO2. Figure 1: N 2 sorption analysis of tetramodal α-MnO 2 . ( a ) N 2 adsorption–desorption isotherms, ( b ) DFT pore size distribution and ( c ) Horvath–Kawazoe pore size distribution from N 2 adsorption isotherm for tetramodal α-MnO 2 . Full size image TEM analysis of tetramodal α-MnO 2 Transmission electron microscopic (TEM) data for tetramodal α-MnO 2 , Fig. 2 , demonstrates a three-dimensional pore structure with a symmetry consistent with space group Ia3d. From the TEM data, an a 0 lattice parameter of 23.0 nm for the mesostructure could be extracted, which is in good agreement with the value obtained from the low-angle powder X-ray diffraction (PXRD) data, a 0 =23.4 nm ( Supplementary Fig. S1a ). High-resolution TEM images in Fig. 2c–e demonstrate that the walls are crystalline with a typical wall thickness of 10 nm. The lattice spacings of 0.69, 0.31 and 0.35 nm agree well with the values of 6.92, 3.09 and 3.46 Å for the [110], [310] and [220] planes of α-MnO 2 (International Centre for Diffraction Data (ICDD) number 00-044-0141), respectively. The wide-angle PXRD data matches well with the PXRD data of bulk cryptomelane α-MnO 2 ( Supplementary Fig. S1b ), confirming the crystalline walls. 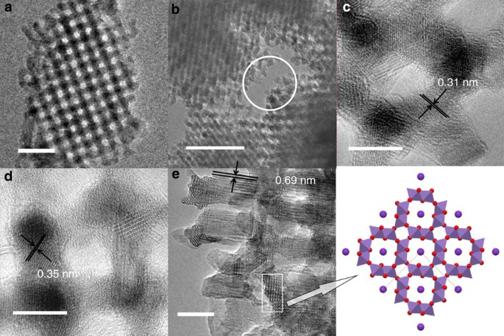Figure 2: TEM images of tetramodal α-MnO2. TEM images along (a) [100] direction, showing 18 nm mesopores (scale bar, 50 nm); (b) 4.0 and 70 nm pores (70 nm pores are highlighted by white circles; scale bar, 100 nm); (c–e) high-resolution (HRTEM) images of tetramodal α-MnO2showing 4.0 and 0.48 nm pores (scale bar, 10 nm). Inset is representation of α-MnO2structure along thecaxis, demonstrating the 2 × 2 micropores as shown in the HRTEM (white box) ine. Purple,octahedral MnO6; red, oxygen; violet, potassium. Figure 2: TEM images of tetramodal α-MnO 2 . TEM images along ( a ) [100] direction, showing 18 nm mesopores (scale bar, 50 nm); ( b ) 4.0 and 70 nm pores (70 nm pores are highlighted by white circles; scale bar, 100 nm); ( c – e ) high-resolution (HRTEM) images of tetramodal α-MnO 2 showing 4.0 and 0.48 nm pores (scale bar, 10 nm). Inset is representation of α-MnO 2 structure along the c axis, demonstrating the 2 × 2 micropores as shown in the HRTEM (white box) in e . Purple,octahedral MnO 6 ; red, oxygen; violet, potassium. Full size image The various pores in tetramodal α-MnO 2 can be observed by TEM directly: the 0.48-nm micropores are seen in Fig. 2e (2 × 2 tunnels with dimensions of 0.48 × 0.48 nm in the white box); the 4.0-nm pores are shown in Fig. 2b–d ; the 18-nm pores are shown in Fig. 2a ; the 70-nm pores are evident in Fig. 2b (highlighted with white circles). Li intercalation Li can be intercalated into bulk α-MnO 2 (ref. 46 ). Therefore, it is interesting to compare Li intercalation into bulk α-MnO 2 (micropores only) and bimodal α-MnO 2 (micropores along with a single mesopore of diameter 3.6 nm, see Methods) with tetramodal α-MnO 2 (micro-, meso- and macropores). Each of the three α-MnO 2 materials was subjected to Li intercalation by incorporation as the positive electrode in a lithium battery, along with a lithium anode and a non-aqueous electrolyte (see Methods). The results of cycling (repeated intercalation/deintercalation of Li) the cells are shown in Fig. 3 . Although all exhibit good capacity to cycle Li at low rates of charge/discharge (30 mA g −1 ), tetramodal α-MnO 2 shows significantly higher capacity (Li storage) at a high rate of 6,000 mA g −1 (corresponding to charge and discharge in 3 min). The tetramodal α-MnO 2 can store three times the capacity (Li) compared with bimodal α-MnO 2 , and 18 times that of α-MnO 2 with only micropores, at the high rate of intercalation/deintercalation ( Fig. 3 ). The superior rate capability of tetramodal α-MnO 2 over microporous and bimodal forms may be assigned to better Li + transport in the electrolyte within the hierarchical pore structure of tetramodal α-MnO 2 . The importance of electrolyte transport in porous electrodes has been discussed recently [35] , [47] , [48] and the results presented here reinforce the beneficial effect of a hierarchical pore structure. 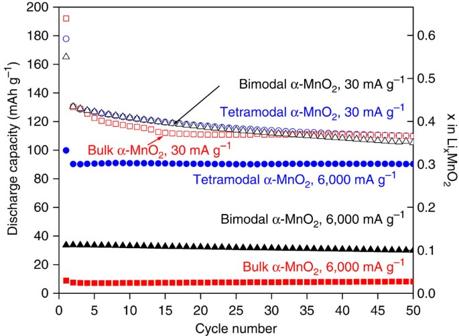Figure 3: Electrochemical behaviour of different α-MnO2. Capacity retention for tetramodal α-MnO2cycled at 30 (empty blue circles) and 6,000 mA g−1(filled blue circles); bulk α-MnO2cycled at 30 (empty red squares) and 6,000 mA g−1(filled red squares); bimodal α-MnO2cycled at 30 (empty black triangle) and 6,000 mA g−1(filled black triangles). Figure 3: Electrochemical behaviour of different α-MnO 2 . Capacity retention for tetramodal α-MnO 2 cycled at 30 (empty blue circles) and 6,000 mA g −1 (filled blue circles); bulk α-MnO 2 cycled at 30 (empty red squares) and 6,000 mA g −1 (filled red squares); bimodal α-MnO 2 cycled at 30 (empty black triangle) and 6,000 mA g −1 (filled black triangles). Full size image Catalytic studies CO oxidation and N 2 O decomposition were used as reactions to probe the three different forms of α-MnO 2 as catalysts ( Supplementary Fig. S2 ). As shown in Supplementary Fig. S2a , tetramodal α-MnO 2 demonstrates better catalytic activity compared with only micropores or bimodal α-MnO 2 ; the temperature of half CO conversion ( T 50 ) was 124 °C for tetramodal α-MnO 2 , whereas microporous and bimodal α-MnO 2 exhibited a T 50 value of 275 °C and 209 °C, respectively. In the case of N 2 O decomposition, α-MnO 2 with only micropores demonstrated no catalytic activity in the range of 200–400 °C, in accord with a previous report [49] . Tetramodal and bimodal α-MnO 2 showed catalytic activity and reached 32% and 20% of N 2 O conversion, respectively, at a reaction temperature of 400 °C. The differences in catalytic activity are related to the differences in the material. A detailed study focusing on the catalytic activity alone would be necessary to demonstrate which specific features of the textural differences (pore size distribution, average manganese oxidation state, K + and so on) between the different MnO 2 materials are responsible for the differences in behaviour. However, the preliminary results shown here do illustrate that such differences exist. Porous LiMn 2 O 4 To demonstrate the wider applicability of the synthesis method, LiMn 2 O 4 with a hierarchical pore structure was synthesized in a way similar to that of tetramodal α-MnO 2 . The main difference is the use of LiNO 3 instead of KNO 3 (see Methods). In this case, Li + reacts with the silica template collapsing/blocking the microporous channels in the KIT-6 and resulting in the large mesopores and macropores (17 and 50 nm) in the LiMn 2 O 4 obtained. The use of Li + instead of the larger K + deters the formation of micropores because Li + is too small. TEM analysis illustrates the hierarchical pore structure of LiMn 2 O 4 ( Supplementary Fig. S3 ): 4.0 nm pores are evident in Supplementary Fig. S3b ; 17 nm pores in Supplementary Fig. S3a ; and 50 nm pores in Supplementary Fig. S3b (highlighted with white circles). The d-spacing of 0.47 nm in the high-resolution TEM image ( Supplementary Fig. S3c ) is in good accordance with the values of 0.4655, nm for the [111] planes of LiMn 2 O 4 (ICDD number 00-038-0789) and with the wide-angle PXRD data ( Supplementary Fig. S4 ). The original DFT pore size distribution analysis from N 2 sorption (adsorption branch) gives three pore sizes in the range of 1–100 nm centred at 4.0, 17 and 50 nm ( Supplementary Fig. S5 ). A more in-depth presentation of the results for LiMn 2 O 4 will be given in a future paper; preliminary results presented here illustrate that the basic method can be applied beyond α-MnO 2 . Turning to the synthesis of the tetramodal α-MnO 2 , the details are given in the Methods section. Hard templating using silica templates, such as KIT-6, normally gives rise to materials with unimodal or, at most, bimodal mesopore structures, and in the latter case the smaller mesopores dominate over the larger mesopores [8] , [32] , [35] . Alkali ions are excellent templates for micropores in transition metal oxides [19] , [21] , but they have been avoided in nanocasting from silica templates because of concerns that they would react with and, hence, destroy the silica template [50] . Here, not only have alkali ions been used successfully in precursor solutions without destroying the template mesostructure but they give rise to macropores in the α-MnO 2 , thus permitting the synthesis of a tetramodal, micro-small, meso-large, meso-macro pore structure. Synthesis begins by impregnating the KIT-6 silica template with a precursor solution containing Mn 2+ and K + ions. On heating, the K + ions template the formation of the micropores in α-MnO 2 , as the latter forms within the KIT-6 template. KIT-6 consists of two interpenetrating mesoporous channels linked by microporous channels [51] , [52] , [53] . The branches of the two different sets of mesoporous channels in KIT-6 are nearest neighbours separated by a silica wall of ~4 nm [53] ; therefore, when both KIT-6 mesochannels are occupied by α-MnO 2 and the silica between them etched away, the remaining pore is 4 nm (see centre portion of Fig. 4 ). It has been shown previously, by a number of authors, that by varying the hydrothermal conditions used to prepare the KIT-6, the proportion of the microchannels can be decreased to some extent, thus making it difficult to simultaneously fill the neighbouring KIT-6 mesoporous channels by the precursor solution of the target mesoporous metal oxide [33] , [34] , [35] . As a result, the target metal oxide grows in only one set of mesochannels of the KIT-6 host but not both. When the KIT-6 is dissolved away, the remaining metal oxide has ~18 nm pores, because the distance between adjacent branches of the same KIT-6 mesochannels is greater than between the two different mesochannels in KIT-6. Here we propose that the K + ions have a similar effect on the KIT-6 to that of the hydrothermal synthesis, but by a completely different mechanism. Reaction between the K + ions in the precursor solution with the silica during calcination results in the formation of K + -silicates, which cause collapse or blocking of the microporous channels in KIT-6, such that the α-MnO 2 grows in one set of the KIT-6 mesochannels, giving rise to 18 nm pores in α-MnO 2 when the silica is etched away, see top portion of Fig. 4 . However, the reaction between K + and the silica is more severe than the effect of varying the hydrothermal treatment. In the former case, the KIT-6 microchannels are so comprehensively destroyed that the proportion of the large (18 nm) to smaller (4 nm) mesopores is greater than can be achieved by varying hydrothermal conditions. The comprehensive destruction of the microchannels in KIT-6 by K + , perhaps augmented by some minor degradation of parts of the mesochannels, leads to α-MnO 2 growing in only a proportion of one set of the KIT-6 mesochannels, resulting in the formation of ~70 nm pores in α-MnO 2 , see lower portion of Fig. 4 . In summary, the K + reactivity with the silica goes beyond what can be achieved by varying the conditions of hydrothermal synthesis and is responsible for generating the tetramodal pore size distribution reported here. 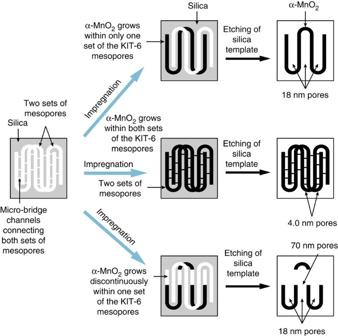Figure 4: Formation mechanism of meso and macropores in tetramodal α-MnO2. When both KIT-6 mesochannels are occupied by α-MnO2and then the silica between them etched away, the remaining pore is 4 nm (centre portion of figure). When α-MnO2grows in only one set of mesochannels and then the KIT-6 is dissolved away, the remaining metal oxide has 18 nm pores (upper portion of figure). The comprehensive destruction of the microchannels in KIT-6 by K+leads to α-MnO2growing in only a proportion of one set of the KIT-6 mesochannels, resulting in the formation of ~70 nm pores (lower portion of figure). Figure 4: Formation mechanism of meso and macropores in tetramodal α-MnO 2 . When both KIT-6 mesochannels are occupied by α-MnO 2 and then the silica between them etched away, the remaining pore is 4 nm (centre portion of figure). When α-MnO 2 grows in only one set of mesochannels and then the KIT-6 is dissolved away, the remaining metal oxide has 18 nm pores (upper portion of figure). The comprehensive destruction of the microchannels in KIT-6 by K + leads to α-MnO 2 growing in only a proportion of one set of the KIT-6 mesochannels, resulting in the formation of ~70 nm pores (lower portion of figure). Full size image The mechanism of pore formation in α-MnO 2 by reaction between K + and the silica template is supported by several findings. First, by the lower K/Mn molar ratio of the final tetramodal α-MnO 2 product (0.08) compared with the starting materials (0.33) implies that some of the K + ions in the impregnating solution have reacted with the silica. Second, support for collapse/blocking of the microporous channels in KIT-6 due to reaction with K + was obtained by comparing the texture of KIT-6 impregnated with an aqueous solution containing only KNO 3 and calcined at 300 and 500 °C. The micropore volume in KIT-6 is the greatest, with no KNO 3 in the solution; it then decreases continuously as the calcination temperature and calcination time is increased, such that after 2 and 5 h at 500 °C the micropore volume has decreased to zero ( Supplementary Fig. S6 ). Third, we prepared tetramodal α-MnO 2 using a similar synthetic procedure to that described in the Methods section, except that this time we used a covered tall crucible for the calcination step. Sun et al. [54] have shown that using a covered, tall crucible when calcining results in porous metal oxides with much larger particle sizes. If the 70-nm pores had arisen simply from the gaps between the particles, then the pore size would have changed; in contrast, it remained centred at 70 nm, Supplementary Fig. S7 , consistent with the 70-nm pores being intrinsic to the materials and arising from reaction with the K + as described above. Fourth, if the synthesis of MnO 2 is carried out using the KIT-6 template but in the absence K + ions, then the DFT pore size distribution shown in Supplementary Fig. S8 is obtained. The 0.48- and 70-nm pores are now absent, but the 4- and 18-nm pores remain. This demonstrates the key role of K + in the formation of the smallest and largest pores and, hence, in generating the tetramodal pore size distribution. The absence of K + means that there is nothing to template the 0.48 nm pores and so α-MnO 2 is not formed; the β-polymorph is obtained instead. The absence of K + also means that the microchannels in the KIT-6 template remain intact, resulting in no 70 nm pores and the dominance of the 4-nm pores compared with the 18-nm pores. The hierarchical pore structure can be varied systematically by controlling the synthesis conditions, in particular the K + /Mn ratio of the precursor solution. A range of K + /Mn ratios, 1/5, 1/3 and 1/2, gave rise to a series of pore size distributions, in which the pore sizes remained the same but the relative proportions of the different pores varied ( Supplementary Table S1 ). The higher the K + /Mn ratio, the greater the proportion of macropores and large mesopores. This is in accord with expectations, as the higher the K + concentration in the precursor solution the greater the collapse/blocking of the microporous channels in the KIT-6 (as noted above), and hence the greater the proportion of macropores and large mesopores. Indeed, these results offer further support for the mechanism of pore size distribution arising from reaction between K + and the silica template. In conclusion, tetramodal α-MnO 2 , the first porous solid with a tetramodal pore size distribution, has been synthesized. Its hierarchical pore structure spans the micro, meso and macropore range between 0.3 and 200 nm, with pore dimensions centred at 0.48, 4.0, 18 and 70 nm. Key to the synthesis is the use of K + ions that not only template the formation of micropores but also react with the silica template, therefore, breaking/blocking the microporous channels in the silica template far more comprehensively than is possible by varying the hydrothermal synthesis conditions, to the extent that macropores are formed, and without destroying the silica mesostructure by alkali ions, as might have been expected. The resulting hierarchical tetramodal structure demonstrates different behaviours compared with microporous and bimodal α-MnO 2 as a cathode material for Li-ion batteries, and when used as a catalyst for CO oxidation and N 2 O decomposition. The method has been extended successfully to the preparation of hierarchical LiMn 2 O 4 . Synthesis Tetramodal α-MnO 2 (surface area 96 m 2 g −1 , K 0.08 MnO 2 ) was prepared by two-solvent impregnation [55] using K + and mesoporous silica KIT-6 as the hard template. KIT-6 was prepared according to a previous report (hydrothermal treatment at 100 °C) [51] . In a typical synthesis of tetramodal α-MnO 2 , 7.53 g of Mn(NO 3 ) 2 ·4H 2 O (98%, Aldrich) and 1.01 g of KNO 3 (99%, Aldrich) were dissolved in ~10 ml of water to form a solution with a molar ratio of Mn/K=3.0. Next, 5 g of KIT-6 was dispersed in 200 ml of n-hexane. After stirring at room temperature for 3 h, 5 ml of the Mn/K solution was added slowly with stirring. The mixture was stirred overnight, filtered and dried at room temperature until a completely dried powder was obtained. The sample was heated slowly to 500 °C (1 °C min −1 ), calcined at that temperature for 5 h with a cover in a normal crucible unless is specified [54] and the resulting material treated three times with a hot aqueous KOH solution (2.0 M), to remove the silica template, followed by washing with water and ethanol several times, and then drying at 60 °C. Bimodal α-MnO 2 (surface area 58 m 2 g −1 , K 0.06 MnO 2 ) with micropore and a single mesopore size of 3.6 nm was prepared by using mesoporous silica SBA-15 as a hard template. The SBA-15 was prepared according to a previous report [56] . Bulk α-MnO 2 (surface area 8 m 2 g −1 , K 0 MnO 2 ) was prepared by the reaction between 325 mesh Mn 2 O 3 (99.0%, Aldrich) and 6.0 M H 2 SO 4 solution at 80 °C for 24 h, resulting in the disproportionation of Mn 2 O 3 into a soluble Mn 2+ species and the desired α-MnO 2 product [46] . Treatment of KIT-6 with KNO 3 was carried out as follows: 1.01 g of KNO 3 was dissolved in ~15 ml of water to form a KNO 3 solution. Five grams of mesoporous KIT-6 was dispersed in 200 ml of n-hexane. After stirring at room temperature for 3 h, 5 ml of KNO 3 solution was added slowly with stirring. The mixture was stirred overnight, filtered and dried at room temperature until a completely dried powder was obtained. The sample was heated slowly to 300 or 500 °C (1 °C min −1 ), calcined at that temperature for 5 h and the resulting material was washed with water and ethanol several times, and then dried at 60 °C overnight. The synthesis method for hierarchical porous LiMn 2 O 4 was similar to that of tetramodal α-MnO 2 . The main difference was to use 1.01 g of LiNO 3 instead of KNO 3 . After impregnation into KIT-6, calcination and silica etching, porous LiMn 2 O 4 was obtained. Characterization TEM studies were carried out using a JEOL JEM-2011, employing a LaB6 filament as the electron source, and an accelerating voltage of 200 keV. TEM images were recorded by a Gatan charge-coupled device camera in a digital format. Wide-angle PXRD data were collected on a Stoe STADI/P powder diffractometer operating in transmission mode with Fe Kα 1 source radiation ( λ =1.936 Å). Low-angle PXRD data were collected using a Rigaku/MSC, D/max-rB with Cu Kα 1 radiation ( λ =1.541 Å) operating in reflection mode with a scintillation detector. N 2 adsorption–desorption analysis was carried out using a Micromeritics ASAP 2020. The typical sample weight used was 100–200 mg. The outgas condition was set to 300 °C under vacuum for 2 h, and all adsorption–desorption measurements were carried out at liquid nitrogen temperature (−196 °C). The original DFT method for the slit pore geometry was used to extract the pore size distribution from the adsorption branch using the Micromeritics software [39] , [40] , [41] , [42] . A Horvath–Kawazoe method was used to extract the microporosity [44] . Mn and K contents were determined by chemical analysis using a Philips PU9400X atomic adsorption spectrometer. The average oxidation state of framework manganese in α-MnO 2 samples was determined by a redox titration method [57] . Electrochemistry First, the cathode was constructed by mixing the active material (α-MnO 2 ), Kynar 2801 (a copolymer based on polyvinylidene fluoride), and Super S carbon (MMM) in the weight ratio 80:10:10. The mixture was cast onto Al foil (99.5%, thickness 0.050 mm, Advent Research Materials, Ltd) from acetone using a Doctor-Blade technique. After solvent evaporation at room temperature and heating at 80 °C under vacuum for 8 h, the cathode was assembled into cells along with a Li metal anode and electrolyte (Merck LP30, 1 M LiPF 6 in 1:1 v/v ethylene carbonate/dimethyl carbonate). The cells were constructed and handled in an Ar-filled MBraun glovebox (O 2 <0.1 p.p.m., H 2 O<0.1 p.p.m.). Electrochemical measurements were carried out at 30 °C using a MACCOR Series 4200 cycler. Catalysis Catalytic CO oxidation was tested in a plug-flow microreactor (Altamira AMI 200). Fifty milligrams of catalyst was loaded into a U-shaped quartz tube (4 mm i.d.). After the catalyst was pretreated in flowing 8% O 2 (balanced with He) at 400 °C for 1 h, the catalyst was then cooled down, the gas stream switched to 1% CO (balanced with air) and the reaction temperature ramped using a furnace (at a rate of 1 °C min −1 above ambient temperature) to record the light-off curve. The flow rate of the reactant stream was 37 cm 3 min −1 . A portion of the product stream was extracted periodically with an automatic sampling valve and was analysed using a dual column gas chromatograph with a thermal conductivity detector. To perform N 2 O decomposition reaction testing, 0.5 g catalyst was packed into a U-shaped glass tube (7 mm i.d.) sealed by quartz wool, and pretreated in flowing 20% O 2 (balance He) at 400 °C for 1 h (flow rate: 50 cm 3 min −1 ). After cooling to near-room temperature, a gas stream of 0.5% N 2 O (balance He) flowed through the catalyst at a rate of 60 cm 3 min −1 , and the existing stream was analysed by a gas chromatograph (Agilent 7890A) that separates N 2 O, O 2 and N 2 . The reaction temperature was varied using a furnace, and kept at 100, 150, 200, 250, 300, 350 and 400 °C for 30 min at each reaction temperature. The N 2 O conversion determined from GC analysis was denoted as X =([N 2 O] in —[N 2 O] out )/[N 2 O] in × 100%. How to cite this article: Ren, Y. et al. A solid with a hierarchical tetramodal micro-meso-macro pore size distribution. Nat. Commun. 4:2015 doi: 10.1038/ncomms3015 (2013).